Out-of-frame start codons prevent translation of truncated nucleo-cytosolic cathepsin Lin vivo The lysosomal protease cathepsin L has been reported to cleave various functionally important cytosolic or nuclear proteins. To explain nucleo-cytosolic localization of cathepsin L, it has been hypothesized that skipping of the first start codon during translation initiation results in an N-terminally truncated protein lacking the endoplasmic reticulum-import signal. Here we demonstrate that out-of-frame AUGs prevent translation of truncated cathepsin L in cell culture as well as in a new knock-in mouse model. We further evaluate potential roles of nuclear cathepsin L during early embryonic development. Our analysis reveals normal epiblast development of cathepsin L-deficient embryos, but uncovers a pronounced lysosomal storage phenotype in the extra-embryonic tissue of the visceral endoderm. In conclusion, the phenotypes of cathepsin L deficiency can be fully assigned to lack of canonically targeted cathepsin L, while the biogenesis and functionality of nucleo-cytosolic cathepsin L remain elusive. Tight regulation of proteolysis is crucial for the maintenance of cellular homoeostasis. Part of this regulation is the correct targeting of proteases to their appropriate cellular compartment. Lysosomal proteases are synthesized as inactive preproenzymes that are targeted into the endoplasmic reticulum (ER) and trafficked via the Golgi apparatus into the lysosome in a mannose-6-phosphate-receptor-dependent manner [1] , [2] . Maturation of the proenzymes takes place in the acidic endosomal/lysosomal compartment, where the proregion is cleaved off autocatalytically or by other lysosomal proteases [3] . However, recent studies discovered cathepsins, the predominant group of lysosomal proteases, in rather unexpected subcellular locations, namely in the cytosol and the nucleus. There these proteases have been proposed to regulate cell proliferation and differentiation (reviewed in ref. 4 ). There are two possibilities under consideration how cathepsins can reach the nucleo-cytosolic compartment. First, they might leak out of the vesicular compartments during the intracellular sorting process or under certain cellular conditions that damage vesicular membranes. However, such leakage from the lysosomal compartment is widely considered as an event that is restricted to cell death [5] , [6] . Second, nucleo-cytosolic cathepsins may not enter the ER at all. For murine cathepsin L, it has been proposed that skipping of the first start codon in translation initiation, termed leaky scanning, leads to N-terminally truncated isoforms, which lack the ER-import signal [7] . Thus, lysosomal targeting is disrupted and translation products remain in the cytosol. Murine cathepsin L and its highly conserved human orthologue cathepsin V (alternatively termed cathepsin L2) are physiologically important proteases and alternative localization would certainly have considerable impact on their function. They are potent ubiquitously expressed endopeptidases with broad substrate specificity that work best at acidic pH and reducing redox conditions [8] , [9] . Cathepsin L-deficient ( Ctsl −/− ) mice reproduce normally, although pups showed a slightly increased mortality during the weaning period [10] . The phenotype of Ctsl −/− mice is characterized by periodical loss of fur hair [10] , [11] , epidermal hyperplasia [10] , [12] , reduced numbers of CD4 + -T cells [13] , [14] and dilated cardiomyopathy in aged animals [15] , [16] . Several studies revealed that cathepsin L affects tumour progression in cancer mouse models [17] , [18] . In addition, cathepsin L is highly overexpressed in several human cancer entities correlating with poor prognosis [19] , [20] , [21] . In the cytosol, cleavage of dynamin, synaptopodin and CD2AP by cathepsin L in renal podocytes leads to cytoskeletal reorganization and triggers the breakdown of the glomerular filtration barrier in a mouse model of proteinuric kidney disease [22] , [23] , [24] . Furthermore, the presence of endogenous cathepsin L inhibitors in the nucleus suggests some degree of regulation of cathepsin L activity in this compartment [25] , [26] . Nuclear cathepsin L has been linked to the regulation of cell proliferation and differentiation. It has been reported to cleave the CDP/Cux transcription factor thereby driving G1/S transition of the cell cycle and by cleavage of 53BP1 cathepsin L might contribute to genomic instability in triple-negative breast cancer cells [7] , [27] , [28] . Nuclear cathepsin L seems to influence histone modifications, since epigenetic marks on the Y chromosome are reorganized in cathepsin L-deficient mouse fibroblasts [29] . Furthermore, recent reports demonstrated cleavage of the N-terminal tail of histone H3 by cathepsin L during embryonic stem (ES) cell differentiation [30] , [31] . This suggests a crucial role of cathepsin L in mouse embryonic development; however, this has not been addressed experimentally yet. Concerning the biogenesis of nuclear or cytosolic cathepsin L, most studies refer to a truncated variant of murine cathepsin L produced by the leaky scanning-based mechanism suggested by Goulet et al . [7] in 2004. However, translational initiation at downstream AUGs is a rather rare event on cellular mRNAs and the regulation of this mechanism is barely understood [32] , [33] . In addition, the current evidence for nuclear cathepsin L functions has been principally obtained by culture approaches, for example, in NIH/3T3 cells, by making use of cathepsin L overexpression constructs. In this study, we focus on the biogenesis of nucleo-cytosolic cathepsin L by closely examining start codon usage in the cathepsin L mRNA in cell culture and - importantly - additionally in vivo . Hence, we established a novel conditional knock-in mouse allele containing a mutated start-AUG thus enforcing alternative translational initiation from the cathepsin L mRNA, while maintaining its physiological transcriptional regulation under the control of the endogenous cathepsin L promotor. Furthermore, we investigated cathepsin L-deficient gastrulation stage embryos for previously unrecognized developmental defects. Our results call the previous hypotheses on biogenesis and functions of nucleo-cytosolic cathepsin L into question. Out-of-frame AUGs stall translation of truncated cathepsin L Translation of the mouse cathepsin L mRNA is initiated after a short untranslated region at the conventional start-AUG in position 83–85 based on the NCBI entry NM_009984.3. This leads to the production of the full-length preprocathepsin L of about 38 kDa molecular weight. After removal of the ER-import signal, the catalytically inactive proform is further processed in the endolysosomal compartment into the active single chain and the fully processed two-chain form of the enzyme [3] . Accordingly, immunoblotting under reducing conditions detects three cathepsin L bands representing the proform (37 kDa), the single-chain form (27 kDa) and the heavy chain of the two-chain form (21 kDa). It has been proposed that skipping of the first start-AUG and usage of downstream start codons results in an N-terminally truncated protein lacking the ER-import signal thus residing in the cytosol or entering the nucleus [7] . Possible alternative translational start sites for a truncated protein would initiate from methionine 56, 58, 75 and 77 based on the amino-acid sequence of the preprocathepsin L (depicted in Fig. 1a as M56, M58, M75, M77, respectively). Close examination of the cathepsin L mRNA showed three additional AUG codons between the conventional start codon M1 and the possible downstream in-frame start codons ( Fig. 1a ). However, usage of these AUGs would lie outside the regular open-reading frame. These alternative AUGs, further termed out-of-frame AUGs (OOF-AUGs), are located at positions 201–203 (OOF-AUG1), 210–212 (OOF-AUG2) and 235–237 (OOF-AUG3) based on the NCBI entry NM_009984.3 ( Fig. 1a ). To estimate the usage of the different AUGs as translation initiation sites, we compared the context of the AUG codons with the Kozak consensus sequence. Here, a guanine following the AUG codon and a purine three nucleotides upstream are highly conserved positions that favour usage as translation initiation sites [34] ( Fig. 1b ). All analysed start codons meet these criteria in one of these positions (underlined characters). Strikingly, the OOF-AUG3 is the only sequence matching the consensus sequence in both positions. Hence, the OOF-AUGs might prevent usage of the downstream in-frame AUGs even in cases where the conventional M1 start codon is skipped. 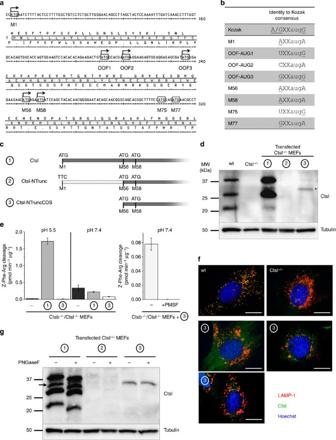Figure 1: Several AUGs have to be skipped to produce an N-terminally truncated cathepsin L variant. (a) Possible translation initiation sites in the mouse cathepsin L mRNA and the corresponding cathepsin L open-reading frame (ORF). NCBI sequence NM_009984.3 with possible translation initiation sites. (b) Identity of the different AUGs to the Kozak consensus sequence. Matches to the Kozak consensus sequence in the conserved sites in −3 and +4 position are marked by underlined characters. (c) Cathepsin L cDNA constructs expressed in Ctsl−/−MEFs: (1) cDNA of full-length cathepsin L, (2) Ctsl-NTrunc cDNA carrying a mutation of M1, (3) Ctsl-NTruncCDS cDNA starting with M56. (d) Cathepsin L immunoblot of Ctsl−/−MEFs transduced with different cathepsin L cDNA variants. Transduction with construct 1 leads to reexpression of full-length cathepsin L. The proform, the single-chain form and the heavy chain of the two-chain form can be seen. No protein derived from construct 2 can be detected. Expression of construct 3 leads to production of a protein of intermediate size (*). (e) Z-Phe-Arg-AMC cleavage assay for Ctsl−/−/Ctsb−/−MEFs transduced with different cathepsin L cDNA constructs. Cleavage of Z-Phe-Arg-AMC at pH 5.5 and 7.4. Aberrant cleavage inCtsl−/−/Ctsb−/−MEFs transduced with construct 3 is fully inhibited by PMSF. Data are presented as mean±s.e.m. (n=3). (f) Immunofluorescence of Ctsl−/−MEFs transduced with the Ctsl-NTruncCDS cDNA construct. Cells were stained for cathepsin L (green), the lysosomal marker LAMP-1 (red) and nuclear staining by Hoechst dye (blue). Expression of construct 3 leads diffuse staining for cathepsin L that does not colocalize with LAMP-1. Scale bar, 10 μm. (g) PNGase-mediated deglycosylation of whole-cell lysates of Ctsl−/−MEFs transduced with different cathepsin L cDNA constructs. All bands seen in the expression of the full-length variant (construct 1) shift on deglycosylation. The protein derived from the Ctsl-NTruncCDS cDNA (construct 3) does not shift on deglycosylation. The band of intermediate size derived from construct 1 shifts on deglycosylation (marked with arrow). Figure 1: Several AUGs have to be skipped to produce an N-terminally truncated cathepsin L variant. ( a ) Possible translation initiation sites in the mouse cathepsin L mRNA and the corresponding cathepsin L open-reading frame (ORF). NCBI sequence NM_009984.3 with possible translation initiation sites. ( b ) Identity of the different AUGs to the Kozak consensus sequence. Matches to the Kozak consensus sequence in the conserved sites in −3 and +4 position are marked by underlined characters. ( c ) Cathepsin L cDNA constructs expressed in Ctsl −/− MEFs: (1) cDNA of full-length cathepsin L, (2) Ctsl-NTrunc cDNA carrying a mutation of M1, (3) Ctsl-NTruncCDS cDNA starting with M56. ( d ) Cathepsin L immunoblot of Ctsl −/− MEFs transduced with different cathepsin L cDNA variants. Transduction with construct 1 leads to reexpression of full-length cathepsin L. The proform, the single-chain form and the heavy chain of the two-chain form can be seen. No protein derived from construct 2 can be detected. Expression of construct 3 leads to production of a protein of intermediate size (*). ( e ) Z-Phe-Arg-AMC cleavage assay for Ctsl −/− /Ctsb −/− MEFs transduced with different cathepsin L cDNA constructs. Cleavage of Z-Phe-Arg-AMC at pH 5.5 and 7.4. Aberrant cleavage in Ctsl −/− /Ctsb −/− MEFs transduced with construct 3 is fully inhibited by PMSF. Data are presented as mean±s.e.m. ( n =3). ( f ) Immunofluorescence of Ctsl −/− MEFs transduced with the Ctsl-NTruncCDS cDNA construct. Cells were stained for cathepsin L (green), the lysosomal marker LAMP-1 (red) and nuclear staining by Hoechst dye (blue). Expression of construct 3 leads diffuse staining for cathepsin L that does not colocalize with LAMP-1. Scale bar, 10 μm. ( g ) PNGase-mediated deglycosylation of whole-cell lysates of Ctsl −/− MEFs transduced with different cathepsin L cDNA constructs. All bands seen in the expression of the full-length variant (construct 1) shift on deglycosylation. The protein derived from the Ctsl-NTruncCDS cDNA (construct 3) does not shift on deglycosylation. The band of intermediate size derived from construct 1 shifts on deglycosylation (marked with arrow). Full size image To test for the effect of the OOF-AUGs and to corroborate that a detectable cathepsin L protein is expressed by translation initiation at codon M56, cathepsin L-deficient ( Ctsl −/− ) mouse embryonic fibroblasts (MEFs) were transduced with different cDNA variants of cathepsin L ( Fig. 1c–g ). We used a full-length variant (construct 1, Fig. 1c ), an M1 point-mutant which still allows usage of all downstream AUGs (Ctsl-NTrunc, construct 2, Fig. 1c ), and the coding sequence (CDS) of a truncated variant starting from M56 (Ctsl-NTruncCDS, construct 3; Fig. 1c ). Immunoblot analysis of whole-cell lysates showed expression of full-length cathepsin L in MEFs transduced with the conventional full-length cDNA (construct 1, Fig. 1c ) but no cathepsin L protein was detected in cells transduced with the M1-mutant construct 2 ( Fig. 1d ). The expression of the Ctsl-NTruncCDS cDNA (construct 3, Fig.1c ) led to the production of a ∼ 30-kDa protein that matches the expected size for the N-terminally truncated variant ( Fig. 1d , marked with *). This confirms that N-terminally truncated cathepsin L can be detected by immunoblotting using our polyclonal antibody. The relative amount of this truncated protein is rather low in comparison with construct 1 expressing the full-length cathepsin L. This is not due to different mRNA expression levels, which are similar for the both constructs ( Supplementary Fig. 1A ). The artificially produced truncated cathepsin L is missing parts of the ERWNIN motif in the propepetide that is known to affect protein folding in closely related cathepsin proteases [35] . Therefore, it is likely that the low levels of truncated cathepsin L are due to misfolding and decreased stability of this protein. To examine proteolytic activity of the cathepsin L variants, we expressed the full-length variant (construct 1) and the truncated variant (construct 3) in cathepsin B and L double-deficient MEFs (see Supplementary Fig. 1B ) and tested cleavage of the prototypical cathepsin B and L peptide substrate z-Phe-Arg-AMC ( Fig. 1e ). High z-Phe-Arg-AMC cleavage at pH 5.5 was obtained by expressing the full-length cathepsin L, while cleavage was absent for the truncated protease. At pH 7.4, some z-Phe-Arg-AMC cleavage was detected, however, this was not correlating with the presence or absence of the cathepsin L variants. Further, the serine protease inhibitor phenylmethylsulphonyl fluoride (PMSF) fully inhibited z-Phe-Arg cleavage in the cells expressing the truncated protein ( Fig. 1e ), indicating that proteases other than the cysteine-type cathepsin L cleave the substrate under neutral conditions. Taken together, the truncated cathepsin L variant is not an active cysteine cathepsin. To check for cellular localization of the truncated protein, we performed immunofluorescence analyses ( Fig. 1f ). In contrast to endogenous cathepsin L, the truncated cathepsin L (generated by expression of Ctsl-NTruncCDS cDNA, construct 3) did not colocalize with the lysosomal marker LAMP-1 (lysosomal-associated membrane protein 1) and showed indeed a rather diffuse cytosolic staining ( Fig. 1f ). Cell fractionation revealed that most of the truncated cathepsin L in the cytoplasm, while only a small amount can be found in the nuclear fraction (see Supplementary Fig. 1C ). To corroborate the direct cytosolic targeting of the truncated cathepsin L, we tested its glycosylation state ( Fig. 1g and Supplementary Fig. 1D ). Glycosylated proteins were captured on a concanavalin A lectin resin (see Supplementary Fig. 1D ). As expected for glycosylated proteins, cathepsin L from wild-type cells as well as from cells expressing full-length cathepsin L derived from construct 1 were strongly enriched in the eluat. The truncated cathepsin L expressed from construct 3 was found exclusively in the flow through, proving the absence of glycosylation on this protein specimen. To test for N-glycosylation, which is only occurring in the lumen of the ER, a PNGase digest to remove N-glycosylations showed clear reduction of the molecular weight in all bands of the full-length cathepsin L (construct 1), while the band of truncated cathepsin L (construct 3) was not shifted ( Fig. 1g ). Together this shows that the artificially produced truncated cathepsin L bypasses the ER import and trafficking through the Golgi. Interestingly, in the PNGase approach ( Fig. 1g ), there is a protein of intermediate molecular weight detected in the lysates of cells transduced with wild-type cDNA (marked by arrow). It has the approximate size of a potential N-terminally truncated cathepsin L variant. However, this band shifted on deglycosylation suggesting that N-glycosylation of this cathepsin L variant had occurred in the ER. Thus, we conclude that leaky scanning biogenesis of this protein specimen is unlikely. The observed protein variant more likely represents an intermediate of cathepsin L processing rather than an N-terminally truncated variant produced by downstream translation initiation. In summary, these experiments show that artificially facilitated translation from the M56 in-frame downstream start codon leads to production of a truncated unglycosylated alternatively localized cathepsin L protein, which is not able to cleave a typical cathepsin L substrate. However, in case of full-length cDNA, it appears that the OOF-AUGs suppress translation of the truncated cathepsin L, as demonstrated by mutating the M1-AUG, which alone was not sufficient to induce usage of downstream in-frame start codons in our cell culture system ( Fig. 1d,g , construct 2). Differential impact of OOF-AUGs To further characterize the effects of OOF-AUGs on repression of translation, we mutated these AUGs in addition to the M1. In three different Ctsl-NTrunc variants, either the first two OOF-AUGs (Ctsl-NTrunc OOF-AUG1+2, construct 4), only the third one (Ctsl-NTrunc OOF-AUG 3, construct 5) or all three (Ctsl-NTrunc OOF-AUG 1+2+3, construct 6) were mutated ( Fig. 2a ). When transduced into Ctsl −/− MEFs, all three cDNAs resulted in comparable expression of cathepsin L mRNA ( Fig. 2b ). When the OOF-AUGs were mutated, we expected to detect a protein of the same size of ∼ 30 kDa as seen for the Ctsl-NTruncCDS variant (construct 3, Fig. 1c,d ). The mutations of OOF-AUGs 1 and 2 did not result in synthesis of any detectable cathepsin L protein ( Fig. 2c , construct 4). When OOF-AUG3 was mutated, small amounts of the truncated variant were detectable ( Fig. 2c , construct 5). Combined mutations of all three OOF-AUGs resulted in abundant synthesis of a readily detectable truncated cathepsin L ( Fig. 2c , comparison of construct 6 and construct 3). In line with the cathepsin L start codon context analysis ( Fig. 1b ), we conclude that the OOF-AUGs, especially the one at position 235–237 (OOF-AUG 3), prevents usage of the downstream in-frame start codons in the cathepsin L mRNA thus hindering translation initiation of truncated cathepsin L in our cell culture system. 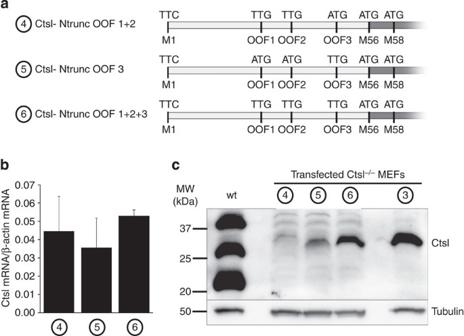Figure 2: Out-of-frame AUGs hinder translation of the truncated cathepsin L variant to a different extent. (a) Cathepsin L cDNA constructs with different mutations in the out-of-frame ATGs: (4) Ctsl-NTrunc ATG-OOF 1+2 carrying a mutation of M1 and ATG-OOF 1 and 2, (5) Ctsl-NTrunc ATG-OOF 3 carrying a mutation of M1 and ATG-OOF 3, (6) Ctsl-NTrunc ATG-OOF 1+2+3 carrying a mutation of M1 and ATG-OOF 1, 2 and 3. (b) mRNA expression of cathepsin L constructs with mutations in out-of-frame AUGs after transduction into Ctsl−/−MEFs. Cathepsin L mRNA expression normalized to β-actin mRNA. Data are presented as mean±s.e.m. (n=3). (c) Immunoblot of Ctsl−/−MEFs transduced with different cathepsin L cDNA constructs with mutations in out-of-frame ATGs. Mutation of ATG-OOF1+2 (construct 4) does not lead to production of a protein of the same size as the one produced by the Ctsl-NTruncCDS construct (construct 3). As soon as the ATG-OOF3 (construct 5) is mutated such a protein is detectable. Combined mutation of all three ATG-OOFs (construct 6) increases the amount of this protein. Figure 2: Out-of-frame AUGs hinder translation of the truncated cathepsin L variant to a different extent. ( a ) Cathepsin L cDNA constructs with different mutations in the out-of-frame ATGs: (4) Ctsl-NTrunc ATG-OOF 1+2 carrying a mutation of M1 and ATG-OOF 1 and 2, (5) Ctsl-NTrunc ATG-OOF 3 carrying a mutation of M1 and ATG-OOF 3, (6) Ctsl-NTrunc ATG-OOF 1+2+3 carrying a mutation of M1 and ATG-OOF 1, 2 and 3. ( b ) mRNA expression of cathepsin L constructs with mutations in out-of-frame AUGs after transduction into Ctsl −/− MEFs. Cathepsin L mRNA expression normalized to β-actin mRNA. Data are presented as mean±s.e.m. ( n =3). ( c ) Immunoblot of Ctsl −/− MEFs transduced with different cathepsin L cDNA constructs with mutations in out-of-frame ATGs. Mutation of ATG-OOF1+2 (construct 4) does not lead to production of a protein of the same size as the one produced by the Ctsl-NTruncCDS construct (construct 3). As soon as the ATG-OOF3 (construct 5) is mutated such a protein is detectable. Combined mutation of all three ATG-OOFs (construct 6) increases the amount of this protein. Full size image Modelling usage of downstream start codons in vivo As translation initiation is complex and the regulation of leaky scanning events that allow usage of alternative start codons might be cell-context dependent, we decided to create an in vivo model for cathepsin L expression from alternative downstream start codons. To resemble the regulation of cathepsin L expression as closely as possible, we employed a knock-in approach in the murine cathepsin L gene to insert a point mutation into the M1-AUG (to TTC) followed by an intronic poly-(A)-signal which acts as a transcriptional stop signal and can be removed by Cre-mediated recombination ( Fig. 3a ). This approach generates a constitutive cathepsin L-null allele with the potential to express an M1-mutated cathepsin L mRNA from the endogenous cathepsin L gene locus. Indeed, after breeding to homozygosity, the mice showed the typical phenotype of the classical constitutive cathepsin L kockout [10] , because the transcriptional STOP cassette terminates transcription in Ctsl intron 2. To induce expression of the M1-mutant cathepsin L mRNA mice harbouring the inactive allele (Ctsl KiTTC STOP ) were bred to mice of the Sox2.Cre general deleter strain, resulting in recombination of the locus (Ctsl KiTTCΔSTOP ) ( Fig. 3b ). In kidney, liver and heart, the levels of cathepsin L mRNA expression from the recombined allele (Ctsl KiTTCΔSTOP ) were comparable with levels of endogenous cathepsin L expression from the wild-type allele ( Fig. 3c ). Sequencing of the mRNA derived from the recombined locus confirmed the expected AUG to TTC mutation in the M1 codon and correct splicing of the mRNA ( Fig. 3d ). Thus, we successfully generated a novel allele for the Ctsl locus, to generate either a null-allele configuration, or to express a cathepsin L mRNA lacking the conventional start codon (M1) under control of the endogenous gene locus. 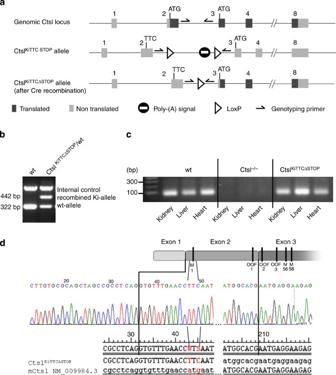Figure 3: Construction of a conditional knock-in for truncated cathepsin L. (a) Schematic of the knock-in approach. By homologous recombination of the knock-in cassette with the mouse cathepsin L locus, the M1 ATG was substituted by TTC. Additionally, the knock-in cassette harboured a poly-A signal in intron 2, which abrogates transcription of the allele (CtslKiTTCSTOP). As this poly-A signal is flanked by LoxP sites, it can be removed by Cre-recombination (results in the recombined allele CtslKiTTCΔSTOP). (b) Genotyping PCR to detect the recombined allele. To activate the knock-in allele, mice were bred with Sox2.Cre mice. Recombination of the knock-in allele was visualized by PCR. Location of the primers is depicted ina. Amplification in the recombined locus leads to a 442-bp PCR product which can be distinguished from the 322-bp product amplified from the wild-type allele. (c) RT–PCR analysis in different organs for cathepsin L mRNA in wild-type (wt), Ctsl−/−and homozygous CtslKiTTCΔSTOP mice. Primers bind in exon 3 and 4 and lead to amplification of a 109-bp PCR product. Expression of cathepsin L mRNA in kidney, liver and heart of homozygous CtslKiTTCΔSTOPmice is comparable with expression in wild-type mice. (d) Sequence of the mRNA derived from the knock-in locus after Cre-recombination. mRNA showed the expected M1 mutation and correct splicing on deletion of the transcriptional STOP cassette. Figure 3: Construction of a conditional knock-in for truncated cathepsin L. ( a ) Schematic of the knock-in approach. By homologous recombination of the knock-in cassette with the mouse cathepsin L locus, the M1 ATG was substituted by TTC. Additionally, the knock-in cassette harboured a poly-A signal in intron 2, which abrogates transcription of the allele (Ctsl KiTTCSTOP ). As this poly-A signal is flanked by LoxP sites, it can be removed by Cre-recombination (results in the recombined allele Ctsl KiTTCΔSTOP ). ( b ) Genotyping PCR to detect the recombined allele. To activate the knock-in allele, mice were bred with Sox2.Cre mice. Recombination of the knock-in allele was visualized by PCR. Location of the primers is depicted in a . Amplification in the recombined locus leads to a 442-bp PCR product which can be distinguished from the 322-bp product amplified from the wild-type allele. ( c ) RT–PCR analysis in different organs for cathepsin L mRNA in wild-type (wt), Ctsl −/− and homozygous CtslKiTTCΔSTOP mice. Primers bind in exon 3 and 4 and lead to amplification of a 109-bp PCR product. Expression of cathepsin L mRNA in kidney, liver and heart of homozygous Ctsl KiTTCΔSTOP mice is comparable with expression in wild-type mice. ( d ) Sequence of the mRNA derived from the knock-in locus after Cre-recombination. mRNA showed the expected M1 mutation and correct splicing on deletion of the transcriptional STOP cassette. Full size image Phenotype of mice expressing M1-mutated cathepsin L The constitutive Ctsl −/− mice have a characteristic gross phenotype as they lose their fur hair in periodical manner dependent on the hair cycle [10] . To test for functional relevance of our novel knock-in allele, we tested if this phenotype could be rescued by expression of N-terminally truncated cathepsin L. However, the loss-of-function hair phenotype was not altered after expression from the knock-in allele ( Fig. 4a ). Furthermore, expression of the mutated cathepsin L mRNA from one allele in combination with the wild-type transcript from the other allele results in a normal appearance as known for Ctsl +/− mice ( Fig. 4a ). In addition to the periodical hair loss, cathepsin L deficiency leads to epidermal hyperproliferation and thickening of the epidermis [10] . Again, expression of the knock-in construct with mutated start-AUG could not rescue the loss-of-function phenotype, and homozygous Ctsl KiTTCΔSTOP/KiTTCΔSTOP animals also showed epidermal thickening ( Fig. 4b ). Furthermore, cathepsin L deficiency disturbs positive selection of CD4 + T cells due to impaired major histocompatibility complex class II complex maturation in thymic epithelial cells leading to reduced numbers of CD4 + /CD8 + cells [13] . Similar to the other cathepsin L loss-of-function phenotypes, this immune phenotype was not further changed by expression of the mutant cathepsin L mRNA and animals showed a similar reduction of CD4 + T-cell number in comparison with Ctsl −/− mice ( Fig. 4c ). 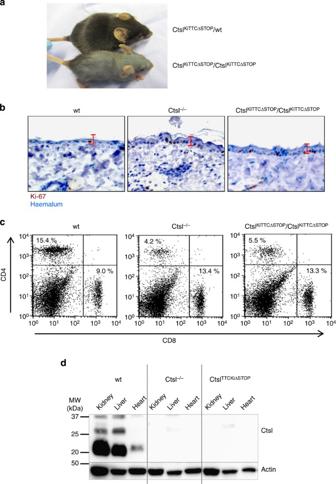Figure 4: Expression of the truncated cathepsin L construct does not rescue the spontaneous phenotypes of cathepsin L-deficient mice. (a) Hair phenotype of mice expressing the knock-in construct. Heterozygous mice carrying one wild-type and one knock-in allele (CtslKiTTCΔSTOP) show no aberrations in normal coat. Homozygous CtslKiTTCΔSTOPmice fully resemble the phenotype of periodical hair loss due to cathepsin L deficiency (littermates; photo taken at p30). (b) Epidermal hyperplasia in wild-type, Ctsl−/−and homozygous CtslKiTTCΔSTOP mice. Paraffin sections of back skin epidermis with Ki67 staining indicating proliferating keratinocytes in the basal layer of the epidermis. In wild-type (wt) epidermis proliferating keratinocytes occur only sporadically. The epidermis in cathepsin L-deficient (Ctsl−/−) mice is thickened and shows numerous proliferating cells. The skin morphology in homozygous CtslKiTTCΔSTOPmice is identical toCtsl−/−. Scale bar, 20 μm. (c) FACS-analysis of the spleen T-cell population in wild-type, Ctsl−/−and homozygous CtslKiTTCΔSTOPmice. Cells were stained for CD4 and CD8 and analysed by flow cytometry. In spleen from wild-type animals∼15% CD4+T cells can be found. Spleens ofCtsl−/−mice show reduced numbers of∼5% CD4+T cells. The amount of CD4+-T cells in the homozygous CtslKiTTCΔSTOPmice were within the same range as in theCtsl−/−. (d) Cathepsin L immunoblot of tissue lysates from different organs in wild-type, Ctsl−/−and homozygous CtslKiTTCΔSTOP mice. There is no cathepsin L protein detectable in kidney, liver and heart lysates of homozygous CtslKiTTCΔSTOPmice. Figure 4: Expression of the truncated cathepsin L construct does not rescue the spontaneous phenotypes of cathepsin L-deficient mice. ( a ) Hair phenotype of mice expressing the knock-in construct. Heterozygous mice carrying one wild-type and one knock-in allele (Ctsl KiTTCΔSTOP ) show no aberrations in normal coat. Homozygous Ctsl KiTTCΔSTOP mice fully resemble the phenotype of periodical hair loss due to cathepsin L deficiency (littermates; photo taken at p30). ( b ) Epidermal hyperplasia in wild-type, Ctsl −/− and homozygous CtslKiTTCΔSTOP mice. Paraffin sections of back skin epidermis with Ki67 staining indicating proliferating keratinocytes in the basal layer of the epidermis. In wild-type (wt) epidermis proliferating keratinocytes occur only sporadically. The epidermis in cathepsin L-deficient ( Ctsl − / − ) mice is thickened and shows numerous proliferating cells. The skin morphology in homozygous Ctsl KiTTCΔSTOP mice is identical to Ctsl − / − . Scale bar, 20 μm. ( c ) FACS-analysis of the spleen T-cell population in wild-type, Ctsl −/− and homozygous CtslK iTTCΔSTOP mice. Cells were stained for CD4 and CD8 and analysed by flow cytometry. In spleen from wild-type animals ∼ 15% CD4 + T cells can be found. Spleens of Ctsl − / − mice show reduced numbers of ∼ 5% CD4 + T cells. The amount of CD4 + -T cells in the homozygous Ctsl KiTTCΔSTOP mice were within the same range as in the Ctsl − / − . ( d ) Cathepsin L immunoblot of tissue lysates from different organs in wild-type, Ctsl −/− and homozygous CtslKiTTCΔSTOP mice. There is no cathepsin L protein detectable in kidney, liver and heart lysates of homozygous Ctsl KiTTCΔSTOP mice. Full size image In summary, the expression of the cathepsin L mRNA that contains a mutation at the conventional start-AUG codon did not induce any gross pathological phenotype in heterozygous animals or rescued the previously described cathepsin L loss-of-function phenotypes. To test for the expression of an N-terminally truncated cathepsin L protein version from our novel knock-in allele, we performed immunoblots of tissues derived from the Ctsl KiTTCΔSTOP mice ( Fig. 4d ). Despite abundant detection of mRNA at similar levels when compared with wild-type alleles ( Fig. 3c ), no expression of cathepsin L protein could be observed in organ lysates from Ctsl KiTTCΔSTOP mice ( Fig. 4d ). These in vivo findings are in line with our cell culture data ( Figs 1 and 2 ) showing that removal of the M1-AUG does not result in sufficient use of alternative in-frame start codons for translation initiation, thus does not result in synthesis of an N-terminally truncated form of cathepsin L. Cathepsin L deficiency in early embryonic development In previous studies, cathepsin L has been reported to cleave the N-terminal tail of histone H3 which contains the majority of modified amino-acid residues that collectively encode for the functional state of histone H3 as chromatin regulator, for example, during ES cell differentiation [30] , [31] . We isolated ES cells using 2i conditions, that is, in presence of inhibitors for MEK and GSK-3 kinases, from wild-type, Ctsl −/− and Ctsl KiTTCΔSTOP mice harbouring the knock-in construct (see Supplementary Fig. 2A ). These ES cell lines were differentiated by omission of the kinase inhibitors and addition of retinoic acid. Within 5 days, all three ES cell lines changed their morphology with the same kinetics to an elongated ‘neuron-like’ appearance ( Supplementary Fig. 2B ) and lost the ES cell marker Oct-3/4 after 2–3 days of differentiation ( Supplementary Fig. 2C ). An N-terminally truncated cathepsin L protein was not produced by the cells harbouring the knock-in allele ( Supplementary Fig. 2C ). We detected a fragment of histone H3 at ∼ 13 kDa. However, this fragment was observed independent of the cathepsin L genotype of the ES cells ( Supplementary Fig. 2C ). To investigate roles of cathepsin L during cell differentiation in vivo at the corresponding embryonic stage, we analysed embryonic day 8.0 (E8.0) Ctsl −/− embryos [36] . Of note, cathepsin L knockout mice are born at the expected Mendelian frequencies and do not show gross phenotypic alterations at birth [10] . However, the close examination of E8.0 Ctsl −/− embryos and control littermates revealed striking morphological differences of the extra-embryonic tissue of the yolk sac of Ctsl −/− embryos. While wild-type yolk sac tissue shows a relatively smooth surface and is translucent, the extra-embryonic yolk sac of the Ctsl −/− embryos exhibits wrinkles and apparent bulging, and was significantly more opaque ( Fig. 5a ). Histological sections of Ctsl −/− embryos further corroborated the malformation of the extra-embryonic visceral endoderm ( Fig. 5b , high magnifications). Although present only transiently during embryogenesis, the visceral endoderm functions in embryonic patterning and nourishing the embryo [37] . Thus, it is characterized by high endocytosis rates and high abundance of acidic endolysosomal vesicles. In line, cathepsin L is strongly expressed in cells of the visceral endoderm as demonstrated by immunohistochemistry of heterozygous control and Ctsl −/− embryos ( Fig. 5c ). Visceral endoderm cells of Ctsl −/− embryos appear considerably enlarged and filled with large vesicular structures staining positive for periodic acid–Schiff and the lysosomal marker LAMP-1 ( Fig. 5d ). This is most likely caused by impaired degradation capacity of the lysosomal compartment representing a lysosomal storage phenotype. Importantly, this morphological alteration does not seem to compromise embryonic development, since the embryo proper does not exhibit any discernable phenotype at early embryonic stages within the epiblast ( Fig. 5a ) and cathepsin L-deficient pubs are born at expected frequency [10] . 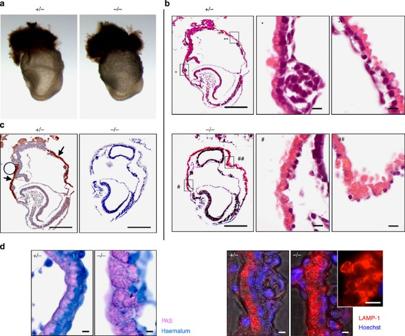Figure 5: Cathepsin L-deficient embryos show no alterations in early development of the epiblast but a severe accumulation of vesicles in the yolk sac endoderm. (a) Morphology of Ctsl−/−embryos in comparison with heterozygous littermates. The yolk sac of cathepsin L-deficient embryos (−/−) is less translucent and exhibits an uneven, bulged surface as compared with heterozygous control littermates (+/−). (b) Paraffin sections of cathepsin L hetero- and homozygous littermates at E8.0 stained by haematoxylin and eosin (HE). Low magnification (Scale bar, 500 μm): the epiblast of the homozygousCtsl−/−embryo (−/−) shows no morphological aberrations. High magnification (Scale bar, 20 μm): heterozygousCtsl+/−embryos (+/−) show a normal structure of the visceral endoderm which is characterized by high endocytotic activity indicated by big vesicular structures (*: anterior, **: posterior part). Embryos deficient for cathepsin L exhibit phenotypic abnormalities in the visceral endoderm, such as wrinkled morphology, thickening of the visceral endoderm cell layer, and increased number and size of vesicular structures. (#: anterior, ##: posterior part). (c) Expression of cathepsin L in E8.0 embryos by immune staining. Cathepsin L is highly expressed in the visceral endoderm of the yolk sac in the heterozygousCtsl+/−embryos, whileCtsl−/−embryos are naturally not stained. Scale bar, 500 μm. (d) Characterization of the vesicles in the visceral endoderm of Ctsl−/−embryos. Left: the vesicular structures of the visceral endoderm in heterozygous (+/−) as well as cathepsin L-deficient (−/−) embryos stain positive for glycoproteins in periodic acid–Schiff (PAS) staining (left panel) as well as for the lysosomal membrane protein LAMP-1 (red) (right panel). The insert shows LAMP-1+vesicles inCtsl−/−embryos at higher magnification. This indicates that the accumulating vesicles are indeed lysosomes. Scale bar, 10 μm. Figure 5: Cathepsin L-deficient embryos show no alterations in early development of the epiblast but a severe accumulation of vesicles in the yolk sac endoderm. ( a ) Morphology of Ctsl −/− embryos in comparison with heterozygous littermates. The yolk sac of cathepsin L-deficient embryos (−/−) is less translucent and exhibits an uneven, bulged surface as compared with heterozygous control littermates (+/−). ( b ) Paraffin sections of cathepsin L hetero- and homozygous littermates at E8.0 stained by haematoxylin and eosin (HE). Low magnification (Scale bar, 500 μm): the epiblast of the homozygous Ctsl − / − embryo (−/−) shows no morphological aberrations. High magnification (Scale bar, 20 μm): heterozygous Ctsl +/ − embryos (+/−) show a normal structure of the visceral endoderm which is characterized by high endocytotic activity indicated by big vesicular structures (*: anterior, **: posterior part). Embryos deficient for cathepsin L exhibit phenotypic abnormalities in the visceral endoderm, such as wrinkled morphology, thickening of the visceral endoderm cell layer, and increased number and size of vesicular structures. (#: anterior, ##: posterior part). ( c ) Expression of cathepsin L in E8.0 embryos by immune staining. Cathepsin L is highly expressed in the visceral endoderm of the yolk sac in the heterozygous Ctsl +/ − embryos, while Ctsl − / − embryos are naturally not stained. Scale bar, 500 μm. ( d ) Characterization of the vesicles in the visceral endoderm of Ctsl −/− embryos. Left: the vesicular structures of the visceral endoderm in heterozygous (+/−) as well as cathepsin L-deficient (−/−) embryos stain positive for glycoproteins in periodic acid–Schiff (PAS) staining (left panel) as well as for the lysosomal membrane protein LAMP-1 (red) (right panel). The insert shows LAMP-1 + vesicles in Ctsl − / − embryos at higher magnification. This indicates that the accumulating vesicles are indeed lysosomes. Scale bar, 10 μm. Full size image An increasing number of functionally important cytosolic or nuclear proteins are assigned as substrates for the lysosomal protease cathepsin L [7] , [22] , [29] , [30] . However, the biogenesis of bona fide cytosolic or nuclear cathepsin L is not well understood. It has been hypothesized that skipping of the first start codon during translation initiation results in an N-terminally truncated cathepsin L variant. This truncated protein is considered to be directly synthesized into the cytosol and able to pass the nuclear membrane by diffusion [7] . Here we report that translation of truncated cathepsin L isoforms is prevented by hindering OOF-AUGs in cells as well as in a targeted mouse model where the first start-AUG was specifically mutated. This novel allele proves that spontaneous phenotypes of cathepsin L-deficient mice can be fully assigned to the lack of canonically targeted cathepsin L. To address the proposed role of cathepsin L as a histone H3-processing enzyme during mouse ES cell differentiation, we performed an early embryonic analysis of cathepsin L-deficient gastrulation stage mouse embryos. Here we observed a pronounced lysosomal storage phenotype in the yolk sac tissue, but fail to find a more general and functionally relevant effect on embryonic development after loss of cathepsin L function. In more detail, transduction of cathepsin L expression constructs in cell culture with either point mutations or deletion of the N terminus revealed that removal of the first canonically used start codon alone was not sufficient to induce translation from downstream in-frame start codons. This is due to three OOF-AUGs located 5′ of the next in-frame start codons, thereby avoiding their usage as translation initiation sites. Especially, the OOF-AUG in position 235–237 (OOF-AUG 3) has a rather strong Kozak context ( Fig. 1b ) and abrogates usage of downstream AUGs. Only on artificial conditions like mutation of the hindering OOF-AUGs or transduction with a cDNA containing exclusively the CDS of the truncated cathepsin L, the corresponding protein was detectable. Thus, translation of native cathepsin L seems to be no exception from the general ‘first-AUG’ rule. However, cell culture experiments may not reflect the situation in vivo. Therefore, we investigated if the translation machinery in vivo is able to skip the OOF-AUGs. A knock-in approach into the genuine cathepsin L locus was chosen as the most physiological approach because all transcriptional and translational mechanisms, which may occur in different cells or tissues, can be correctly executed in this model. As the first cathepsin L start codon M1 was mutated, the mRNA can be more easily used for translation initiation at any downstream start codon. However, the mutation of the canonical M1-AUG codon resulted in a complete lack of any cathepsin L protein synthesis despite abundant mRNA expression. Thus, we conclude that skipping of the first translational start-AUG is unlikely to account for a general mechanism for the generation of an N-terminally truncated cathepsin L protein version in vivo . Consequently, the expression of the M1-mutated cathepsin L transcript fails to rescue the described cathepsin L knockout phenotypes, such as the periodic loss of hair, epidermal hyperplasia as well as the impaired positive selection of CD4 + -T cells. Accordingly, we conclude that the phenotypes of cathepsin L-deficient mice can be assigned to the lack of canonically targeted cathepsin L. The scope of this study was to address the biogenesis of truncated cathepsin L under physiological conditions in healthy mice. Yet it cannot be excluded that leaky scanning-derived truncated cathepsin L forms may be translated and functionally important on pathological conditions such as cancer, or inflammation. However, leaky scanning is considered to be strongly dependent on a permissive mRNA-sequence context in proximity to the potential start codons, and, to date, little is known about how external factors might regulate differential start codon usage [32] , [33] . Thus, our results strongly suggest that the three OOF-AUGs efficiently hinder murine cathepsin L translation initiation from downstream in-frame start codons independent of the functional state of cells and tissues. However, alternative possibilities for the generation of truncated nonvesicular cathepsin L isoforms could be envisioned. For example, the formation of an internal-ribosomal-entry-site structure could enable ribosomal entry directly at the downstream in-frame AUG. However, the existence of such mechanisms for cellular mRNAs is still under discussion [32] , [38] . Alternatively, a mechanism relying on the production of a different cathepsin L mRNA species might be more liable. For human cathepsin B, a splice variant that lacks the exon 2 has been described [39] , [40] . In general, alternative splicing would also be possible for mouse cathepsin L. However, such a splice variant would still contain the OOF-AUG 2 and 3 which are located in exon 3 together with the downstream in-frame start codons (see Fig. 3d ). A third option would be the production of a shorter transcript by usage of an alternative downstream promoter as described for other mRNAs [41] , [42] . However, all transcriptional and translational mechanisms could still be executed on our novel allele with the M1-mutated locus. This would in all cases result in the production of a non-glycosylated cathepsin L protein of intermediate size. Nevertheless, we have never been able to detect such a truncated unglycosylated cathepsin L protein. Besides these mechanisms based on N-terminally truncated variants, one should reconsider nucleo-cytosolic cathepsin L derived from low-level lysosomal permeabilization or retrograde protein trafficking of the conventional full-length protein [43] , [44] . In conclusion, our data do not support the current hypothesis of biogenesis of nucleo-cytosolic cathepsin L. To functionally address the role of nucleo-cytosolic cathepsin L, we investigated the proposed role of nuclear cathepsin L as a histone H3-processing enzyme during ES cell differentiation in ES cells derived from our novel knock-in strain and by analysing the early development of Ctsl −/− embryos. First, there were no differences between the various cathepsin L genotypes when ES cells undergo differentiation and a cathepsin L-dependent histone H3 clipping was not observed. Second, the epiblast-derived embryo showed no morphological aberrations. In summary, these data exclude crucial functions of cathepsin L-mediated histone H3 cleavage events during early mouse development. Instead, we uncovered a striking phenotype in the visceral endoderm of the extra-embryonic yolk sac showing large lysosomal accumulations. Similar vesicular accumulations have already been found in MEFs, keratinocytes and cardiomyocytes of Ctsl −/− mice [11] , [15] , [45] , [46] . Most likely these vesicular accumulations represent a variation of classical storage disorders triggered by impaired lysosomal degradation [47] . This additional phenotype supports the importance of cathepsin L in lysosomal degradation. Interestingly, the visceral endoderm phenotype in mice resembles findings in cathepsin L protease-deficient Caenorhabditis elegans embryos, where ablation of cathepsin L leads to a lethal accumulation of yolk platelets [48] , [49] . In mice, the endoderm of the yolk sac contributes to nutrition of the embryo by providing nutrients obtained from endocytosed material [37] . Observed disturbances on cathepsin L deficiency might impair the nutrient supply, possibly contributing to the slightly increased mortality of cathepsin L-deficient pups during the weaning period [10] . Finally, one might revisit the view on cathepsin L functions in the cytosol or in the nucleus. Certain effects observed on cathepsin L deletion or inhibition might be due to downstream effects of impaired endosomal–lysosomal functionality rather than direct cleavage events. For instance, cathepsin L effects proliferation by its role in endolysosomal termination of mitogenic signalling by degradation of growth factors and their receptors [12] , [50] . Furthermore, it has been shown that deficiency of cathepsins leads to altered expression of several proteases and protease inhibitors leading to additional downstream effects in the cell [51] due to overall changes in the proteolytic network [52] , [53] . In summary, we show that leaky scanning on the mouse cathepsin L mRNA is unlikely to be a physiological mechanism to produce an N-terminally truncated nucleo-cytosolic cathepsin L isoform. Thus, the conditions for the biogenesis of bona fide nucleo-cytosolic cathepsin L are still open to further investigation. Animals Generation of conditional knock-in mice: the murine cathepsin L ( Ctsl ) gene was targeted by homologous recombination in C57BL/6N ES cells for constitutive replacement of the first ATG (Met) translation initiation site by TTC (Phe) and the insertion of a loxP-flanked transcriptional STOP (Poly-A signal) cassette along with an frt-flanked puromycine resistance cassette into Ctsl intron 2. From 273 resistant clones, 32 correctly targeted clones were identified by PCR. Five ES cell clones were further validated by Southern blot and long-range PCR. Two clones were microinjected into BALB/c blastocysts and transferred into pseudopregnant NMRI mice. Highly chimeric offspring mice were mated with female C57BL/6 mice transgenic for Flp-recombinase to remove the frt-flanked resistance marker. Removal of the loxP-flanked STOP cassette for expression of the cathepsin L mRNA lacking the regular start codon was achieved by breeding to the general deleter strain SOX2.Cre [54] . Primers flanking the STOP cassette in Ctsl intron 2 (CLKi-forward: 5′- CCAATCATACATCCATTG-TGAGC -3′, CLKi-reverse: 5′- GGGTTTCTTTTCTGTATAGCTCAGG -3′) allowed for differentiation of the wild type and loxP site containing alleles after deletion of the STOP cassette. PCR amplification of the CD79b gene locus by the primer pair Ctrl forward: 5′- GAGACTCTGGCTACTCATCC -3′/Ctrl reverse: 5′- CCTTCAGCAAGAGCTGGGGAC -3′ served as internal control. The generation of the constitutively Ctsl − / − mice has been described previously [10] . Mouse work in this study was approved by the ethics committee of regional council Freiburg (ethics approval registration number G-07/26 RP Freiburg) and performed in accordance to the German law for animal protection (Tierschutzgesetz) as published on 25 May 1998. Cell culture and stable transduction MEFs were prepared as described previously [45] . Briefly, embryos of the genotypes wild type, Ctsl − / − and Ctsb − / − Ctsl − / − were killed at embryonic day 12.5. The head and internal organs were removed, and the torso was minced and dispersed in 0.25% trypsin (Gibco/Invitrogen, Paisley, UK) for 15 min at 37 °C. Cells were cultured in Dulbecco’s modified Eagle’s medium (Gibco/Invitrogen) supplemented with 10% fetal calf serum (PAN, Aidenbach, Germany) 1% penicillin/streptomycin and 2 mM L-glutamine (both from Gibco/Invitrogen) in humidified air containing 5% CO 2 . Cells were spontaneously immortalized by repeated passaging for at least 25 passages. For the expression of different cathepsin L cDNAs cells were stably transfected by lentiviral transduction, employing the pMISSION system (Sigma-Aldrich, St Louis, MO, USA) as previously described [55] . ES cell culture and differentiation ES cells were isolated as described using 2i medium conditions [56] . In brief, E3.5 blastocysts were isolated after timed mating by flushing of the uterus horns with M2 medium (Sigma). Blastocysts were transferred in 96-well plates onto mitose-inhibited MEFs in 2i ES cell medium (500 ml high-glucose Dulbecco’s modified Eagle’s medium (Gibco/Invitrogen), 15% fetal bovine serum (Gibco/Invitrogen), 1% L -glutamine (Gibco/Invitrogen), 1% sodium-pyruvate (Gibco/Invitrogen), 1% nonessential amino acids (Gibco/Invitrogen), 1% penicillin/streptomycin (Gibco/Invitrogen), 0.1 mM ß-mercaptoethanol (Sigma), 1 μM MEK inhibitor PD0325901 (AxonMedchem, Groningen, The Netherlands), 3 μM GSK-3 inhibitor CHIR99021(AxonMedchem). On day 5 after plating the cells from the outgrowth of the inner cell mass were trypsinized and replated onto MEFs in 24-well format. Following splits were done according to cell density every other day using gelatinized plates without MEF feeder cells. 2i medium was changed daily. Feeder-free ES cells were genotyped after six passages and used for further experiments. For differentiation, cells were seeded on gelatinized plates in ES cell medium without the two inhibitors and addition of 0.1 μM retinoic acid (Sigma). DNA cloning The cathepsin L cDNA was cloned into the pLHCX expression vector (Clontech, Mountain View, CA, USA) via Hin dIII and Cla I using primers flanking either the whole CDS or the downstream sequence starting with M56. Site-directed mutagenesis to delete ATG sites was performed according to the manufacturer’s instructions (Quick Change II, Agilent, Santa Clara, CA, USA). RT–PCR and qPCR analysis RNA was isolated from tissues and cells using the RNeasy Mini Kit (Qiagen, Hamburg. Germany) and transcribed to cDNA using the iSCRIPT cDNA synthesis system (Bio-Rad, Hercules, CA, USA). Primer sequences for reverse transcriptase–PCR (RT–PCR) or quantitative real-time PCR were as follows: Ctsl forward 5′- GCACGGCTTTTCCATGGA -3′; Ctsl reverse: 5′- CCACCTGCCTGAATTCCTCA -3′; β-actin forward: 5′- ACCCAGGCATTGCTGACAGG -3′; β-actin reverse: 5′- GGACAGTG AGGCCAGGATGG -3′. Quantitative RT–PCR was performed using Platinum SYBR Green qPCR SuperMix-UDG (Life Technologies, Darmstadt, Germany) and PCR was run in the CFX96 real-time PCR machine (Bio-Rad). RT–PCR products were analysed on a sodium-borate buffered 1% agarose gel. Preparation of protein lysates Organs from 8–10-week-old male animals were harvested after perfusion with 0.9% NaCl and 0.4 units ml −1 heparin. Fresh tissue samples ( ∼ 100 mg) were lysed in 1 ml of homogenization buffer (100 mM Na acetate, 5 mM EDTA, 1 mM dithiothreitol (DTT), 0.05% Brij, pH 5.5 and protease inhibitor (Complete inhibitor cocktail, Roche, Basel, Switzerland)) using an Ultra-Turrax and debris was pellet at 1,000 g for 15 min at 4 °C. Whole-cell lysates were prepared by on-plate lysis. Cells were washed with PBS and lysed by adding lysis buffer containing 50 mM Tris-HCl (pH 8), 250 mM NaCl, 2.5 mM EDTA, 2% Nonident-P-40, 0.1% SDS, 0.5% sodium-deoxycholate and protease inhibitors (Complete inhibitor cocktail). For cytoplasmic and nuclear fractions, cells were lysed in 50 mM Tris-HCl (pH 7.6), 150 mM NaCl, 5 mM MgCl 2 0.1% NP-40, 1 mM E64, 1 mM PMSF, 1 mM Pefabloc and incubated on ice for 30 min. Nuclei were pelleted at 13,000 g and dissolved in SDS-loading buffer, whereas the supernatant was used as cytoplasmic lysate. Protein concentrations were determined by bicinchoninic acid assay (Thermo Scientific, Waltham, MA, USA). Enrichment of glycosylated proteins and PNGase digest To enrich for glycosylated proteins, whole-cell lysates in PBS, 1% Triton-X 100, 1 mM E64, 1 mM PMSF, 1 mM Pefabloc were used according to the manufacturer’s protocol (Glycoprotein Isolation Kit, concanavalin A, Thermo Scientific). For deglycosylation, protein lysates were pretreated with PNGaseF according to the manufacturer’s protocol (New England Biolabs, Hitchin, UK). Immunoblot In total, 10–40 μg of lysate was loaded onto 12% SDS–polyacrylamide gels. After electrophoretic separation, proteins were transferred on polyvinylidene fluoride membranes by semidry blotting (Bio-Rad). After blocking with 3% milk powder in PBS with 0.1% Tween, the membranes were exposed to the primary antibodies (polyclonal goat-α-mouse cathepsin L 1:500 (catalogue no. AF1515, R&D Systems, Minneapolis, MN, USA), mouse-α-mouse tubulin 1:1,000 (catalogue no. T6199, Sigma-Aldrich, Hamburg, Germany) mouse-α-mouse actin 1:1,000 (catalogue no. 691001, MP Biomedicals, Solon, OH, USA), polyclonal rabbit-α-mouse histone H3 1:1,000 (catalogue no. ab1791, Abcam, Cambridge, UK), mouse monoclonal α-mouse/human Oct-3/4 (catalogue no. sc-5279, Santa Cruz Biotechnology, Dallas, TX, USA) overnight at 4 °C. Membranes were washed and incubated for 2 h with the respective secondary antibody (rabbit-α-goat IgG-POD (catalogue no. A5420) and goat-α-mouse IgG-POD (catalogue no. A4416), both Sigma-Aldrich). Membranes were washed and developed with the West Femto Chemiluminescent substrate (Pierce, Rockford, IL, USA). Light emission was detected using the Fusion SL Detection System (Peqlab, Erlangen, Germany). Enzyme activity assay Cells were lysed by on-plate lysis in 200 mM sodium acetate (pH 5.5), 1 mM EDTA, 0.05% Brij, 1 mM DTT for activity under acidic conditions. For activity measurements under neutral conditions, cell lysis was performed in 50 mM Tris (pH 7.5), 25 mM KCl, 10 mM NaCl, 1 mM MgCl 2 , 0.5 mM DTT, 0.05% NP-40. Additionally, cells were disrupted by ultrasound. In respective samples, the serine protease inhibitor PMSF was added to 1 mM and samples were heated up to 37 °C before the addition of the fluoropeptide z-Phe-Arg-4-methyl-coumarin-7-amide (Bachem, Torrance, CA, USA) to an end concentration of 0.5 nM. The release of 7-amino-4-methyl-coumarin was measured every minute over a time period of 45 min at excitation and emission wavelengths of 360 and 460 nm, respectively. Enzyme activity was normalized to protein concentration. Immunofluorescence staining Cells were seeded on glass coverslips in 24-well plates. Next day, cells were washed with PBS, fixed with 4% paraformaldehyde (PFA) at 37 °C for 30 min and permeabilized with 0.2% Triton-X 100 (diluted in PBS) at room temperature (RT) for 7 min and with acetone at −20 °C for 4 min. A blocking step was performed using 2.5% bovine serum albumin (BSA) for 30 min at RT. Incubation with primary antibodies rat-α-mouse LAMP-1 (catalogue no. 25245, 1:750, Abcam, Cambridge, UK) and polyclonal goat-α-mouse cathepsin L 1:500 (catalogue no. AF1515, R&D Systems, Minneapolis, MN, USA) was performed at 4 °C overnight and incubation with secondary antibodies (goat-α-rat IgG Alexa Fluor 594 and donkey-α-goat IgG Alexa Fluor 488 (Life Technologies)) was performed at RT for 1 h. Nuclear counterstain was performed with Hoechst (Sigma-Aldrich, 2 μg ml −1 in PBS) at RT for 5 min and coverslips were mounted with Permaflour (Thermo Scientific). Images at × 1,000 magnification (× 100 PlnN 1.3 oil objective) were taken using a Zeiss Observer.Z1 fluorescence microscope (Carl Zeiss, Oberkochen, Germany) at 475(ex)/530(em) nm for green fluorescence, 530–585(ex)/615(em) nm for red fluorescence and 365(ex)/445–450(em) nm for blue fluorescence. Images were taken with an AxioCam MRm camera (Carl Zeiss) and processed with the Axio Vision software (Carl Zeiss). Histological analysis of the skin and embryos Pieces of dorsal skin were fixed in PFA and processed for paraffin embedding. A total of 10-μm paraffin sections of back skin were deparaffinized, blocked with 2.5% BSA and 1.5% rat serum, and incubated with the primary antibody (catalogue no. M7249, rat-α-mouse Ki67, Dako, Glostrup, Denmark). Embryos were dissected at embryonic day E8.0, fixed in 4% PFA, dehydrated through an ethanol series and embedded in paraffin before sectioning at 8 μm. Sections were deparaffinized and stained with hematoxylin and eosin or blocked with 2.5% BSA and 1.5% rat serum for 30 min at RT and incubated with cathepsin L antibody overnight at 4 °C (1:500, catalogue no. AF1515, R&D Systems, Minneapolis, MN, USA). Antibody detection on skin and embryo sections was visualized using the Vectastain Elite ABC Kit (Vector Laboratories, Burlingame, CA, USA). Periodic acid–Schiff staining was performed on paraffin sections according to the manufacturer’s protocol (Carl Roth, Karlsruhe, Germany). For immunofluorescence staining, cryosections were prepared according to standard protocols [57] . LAMP-1 staining was performed as described for cell staining on coverslips. Images were collected on an Axioplan microscope (Zeiss, Stuttgart, Germany). Adobe Photoshop software was used for moderate contrast enhancement. Analysis of the T-cell population by flow cytometry Spleens were dissected from 8-week-old animals and passed through a 100-μm cell strainer. Cells were washed with PBS once and incubated in erythrocyte lysis buffer (0.15 M NH 4 Cl, 1 mM KHCO 3 and 0.1 M EDTA in double-distilled H 2 O) for 5 min on ice. Cells were washed twice with FACS-buffer (2% FCS in PBS). In total, 1 × 10 6 cells were incubated with rat-α-mouse CD4 PE and rat-α-mouse CD8a APC (both BD Biosciences, Heidelberg, Germany) or the respective isotype control for 30 min on ice. Cells were measured using the FACScalibur (BD Biosciences) and data were analysed with Cell Quest Software (BD Biosciences). How to cite this article : Tholen, M. et al . Out-of-frame start codons prevent translation of truncated nucleo-cytosolic cathepsin L in vivo . Nat. Commun. 5:4931 doi: 10.1038/ncomms5931 (2014).